Netrin-dependent downregulation of Frazzled/DCC is required for the dissociation of the peripodial epithelium inDrosophila Netrins are secreted chemoattractants with roles in axon guidance, cell migration and epithelial plasticity. Netrin-1 also promotes the survival of metastasized cells by inhibiting the pro-apoptotic effects of its receptor Deleted in Colorectal Carcinoma (DCC). Here we report that Netrins can also regulate epithelial dissociation during Drosophila wing eversion. During eversion, peripodial epithelial cells lose apico-basal polarity and adherens junctions, and become migratory and invasive—a process similar to an epithelial–mesenchymal transition. Loss of netrinA inhibits the breakdown of cell–cell junctions, leading to eversion failure. In contrast, the Netrin receptor Frazzled blocks eversion when overexpressed, whereas frazzled RNAi accelerates eversion in vitro . In peripodial cells Frazzled is endocytosed, and undergoes NetA-dependent degradation, which is required for eversion. Finally, we provide evidence that Frazzled acts through the ERM-family protein Moesin to inhibit eversion. This mechanism may also help explain the role of Netrin and DCC in cancer metastasis. Epithelial–mesenchymal transitions (EMTs), the process by which epithelial cells dissociate and become migratory, are a key mechanism in development, tissue regeneration and disease [1] , [2] . EMTs typically involve loss of epithelial apico-basal polarity and adhesive cell–cell junctions, and the acquisition of cell motility and invasiveness accompanied by breakdown of extracellular basement membranes. In animals, EMTs occur at several stages of development such as gastrulation, neural crest formation and in later events such as the formation of the heart valve and secondary palate [3] . As molecular mechanisms regulating developmental EMTs also occur in cancer metastasis, there has been renewed interest in in vivo models of EMT [4] . In spite of this, relatively few genes regulating EMT have been identified in a key genetic model organism, Drosophila melanogaster . In flies, two important developmental EMTs occur during gastrulation with the formation of the mesoderm and endoderm. The mesodermal EMT is induced by the transcription factors Twist, a master regulator of mesodermal cell fate, and Snail, a repressor of the epithelial adhesion molecule E-Cadherin (E-Cad) [5] , and also involves the combined actions of cell division and the fibroblast growth factor receptor Heartless [6] . For the endodermal EMT, the GATA-factor Serpent downregulates E-Cad through repression of the polarity factor Crumbs [7] . As human orthologues of Twist, Snail, E-Cad and Serpent are strongly associated with metastatic cancers, the identification of new EMT factors in the fly is of great interest. To find new factors regulating EMT, we conducted an RNA interference (RNAi) screen for genes required for an EMT-like event that occurs during pupal metamorphosis: the eversion of wing imaginal discs. Imaginal discs are flattened epithelial sacs attached to the inside body wall of the larva, which proliferate and are patterned during larval development. They consist of a columnar ‘disc proper’ epithelium on one side that gives rise to adult structures such as the thorax and wing and a thin, squamous, peripodial epithelium whose basal surface comes into apposition with the larval epidermis. During eversion, activation of the Jun kinase (JNK) signalling pathway in peripodial cells induces expression of matrix metalloproteases (MMPs), which degrade the basement membrane that lies between the periopodial epithelium and the epidermis [8] . Peripodial cells lose apico-basal polarity, delocalize cell–cell adhesion molecules such as E-Cad and extend F-actin-rich protrusions as they invade, and then migrate over, the epidermal cells as an epithelial sheet [9] . Eventually, disc cells from left and right sides meet at the dorsal midline and fuse to form the pupal/adult epithelium. Failure of eversion leads to adult phenotypes such as internalized wings and missing thoracic tissue [8] . In our screen, we identified the secreted chemoattractant NetrinA. In this study, using live imaging we show that netrinA ( netA ) knockdown in peripodial cells inhibits the ability of wing discs to break through the larval epidermis and evert. Using a wing disc culture assay [10] , we then show that loss of netrins inhibits the dissolution of zonula adherens (ZA) and formation of holes in the peripodial epithelium. We find that netrins promote eversion by downregulating the Deleted in Colorectal Carcinoma (DCC)-family receptor Frazzled (Fra), as loss of netrins increases levels of Fra and reducing Fra levels rescues netrin eversion defects and accelerates the ZA fragmentation and formation of holes. The molecular pathway by which Fra inhibits epithelial dissociation appears to include the ERM-family protein Moesin (Moe), as Fra promotes phosphorylation of Moe, and knockdown of moesin rescues netrin eversion defects. Netrins regulate many cellular processes [11] but have not previously been shown to promote epithelial breakdown. Given the importance of EMT in cancer metastasis, our findings raise the possibility that the role of Netrins and their receptors in metastasis may extend beyond regulation of apoptosis [12] , [13] . netA is required for wing disc eversion Using the peripodial driver, Ubx-GAL4 , we screened UAS inverted repeat (IR) RNAi libraries for genes that were required for eversion. 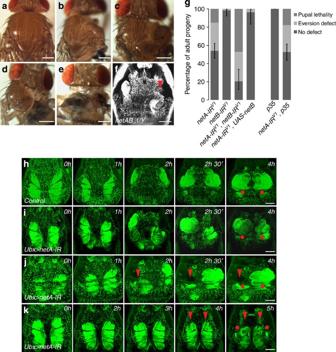Figure 1: Netrin is required forDrosophiladisc eversion. (a)Ubx-GAL4/+control fly. (b–e)netA-IRfly phenotypes including twisted thorax and crumpled wing tissue (b), thoracic cleft (c), single-sided eversion failure with internalized adult wing visible and loss of associated thoracic tissue (d) and double-eversion failure with both wings internalized and no external thoracic tissue (e). (f) DissectednetABΔ/Y pupae, ~4.5 h after puparium formation. A single disc has everted while the second disc remains internalized (arrowhead). Nuclei are marked using Hoechst 33258. (g) Penetrance of defects generated by alterednetAandnetBexpression. The three categories are: ‘no defect’—which includes both eclosed and pharate adults with normal wings and thorax, ‘eversion defect’—which includes defects shown inb–e. ‘Pupal lethality’—where pupae died before adult eversion phenotypes could be assayed. For each genotype,n>50 progeny were scored (seeTable 1). Error bars show 95% confidence intervals (Wilson score method) for the proportion with no defect. (h–k) Live imaging of controlUbx-GAL4/+(h) andUbx>netA-IR(i–k) pupae expressing the nuclear markerHis2Av-EGFP. (h) Control sequence in which wing imaginal discs move laterally (1 h), break through the epidermis (2 h), migrate together (2 h 30') and meet at the midline. (i) AUbx>netA-IRpupa in which both discs evert, but the thorax closure process is abnormal. (j) AUbx>netA-IRpupa in which a single disc fails to evert (red arrowhead). (k) AUbx>netA-IRpupa where both discs fail to evert. Note that haltere discs (red asterisks) always everted. Scale bars, 200 μm (a–f,h–k). RNAi knockdown of netA using the UAS-netA-IR V1 line (see Table 1 for stock nomenclature) disrupted normal eversion ( Fig. 1a ) resulting in a range of phenotypes including internalized wings and missing thoracic tissue (14.5%, n =180; Fig. 1d,e ), crumpled wings (6.1%; Fig. 1b ), thoracic clefts (10.6%; Fig. 1c ) and early pupal lethality (15%; Fig. 1g ). Knockdown of the functionally redundant netA paralogue, netB [14] , [15] , also resulted in low penetrance eversion defects (1.3% n =229, for UAS-netB-IR V1 ). Eversion defects were also observed with two other netA RNAi lines, and an independent RNAi line to netB ( Table 1 ). Combined RNAi to netA and netB increased early lethality to 44.8% ( n =143) and eversion defects to 32.9%. Strikingly, co-expression of a netB transgene, which should not be targeted by the RNAi, reduced Ubx>netA-IR V1 ( netA-IR) phenotypes to only 8.6% ( n =70; Fig. 1g ). Table 1 Adult disc eversion defects generated by netA knockdown. Full size table Figure 1: Netrin is required for Drosophila disc eversion. ( a ) Ubx-GAL4/+ control fly. ( b – e ) netA-IR fly phenotypes including twisted thorax and crumpled wing tissue ( b ), thoracic cleft ( c ), single-sided eversion failure with internalized adult wing visible and loss of associated thoracic tissue ( d ) and double-eversion failure with both wings internalized and no external thoracic tissue ( e ). ( f ) Dissected netAB Δ /Y pupae, ~4.5 h after puparium formation. A single disc has everted while the second disc remains internalized (arrowhead). Nuclei are marked using Hoechst 33258. ( g ) Penetrance of defects generated by altered netA and netB expression. The three categories are: ‘no defect’—which includes both eclosed and pharate adults with normal wings and thorax, ‘eversion defect’—which includes defects shown in b – e . ‘Pupal lethality’—where pupae died before adult eversion phenotypes could be assayed. For each genotype, n >50 progeny were scored (see Table 1 ). Error bars show 95% confidence intervals (Wilson score method) for the proportion with no defect. ( h – k ) Live imaging of control Ubx-GAL4/+ ( h ) and Ubx>netA-IR ( i – k ) pupae expressing the nuclear marker His2Av-EGFP . ( h ) Control sequence in which wing imaginal discs move laterally (1 h), break through the epidermis (2 h), migrate together (2 h 30') and meet at the midline. ( i ) A Ubx>netA-IR pupa in which both discs evert, but the thorax closure process is abnormal. ( j ) A Ubx>netA-IR pupa in which a single disc fails to evert (red arrowhead). ( k ) A Ubx>netA-IR pupa where both discs fail to evert. Note that haltere discs (red asterisks) always everted. Scale bars, 200 μm ( a – f,h – k ). Full size image As loss of vertebrate Netrin-1 can result in DCC-dependent apoptosis, we tested whether eversion defects might be due to excessive cell death. However, neither the defects associated with netA RNAi or fra overexpression were affected by co-expression of the caspase inhibitor p35 ( Fig. 1g and see below). The dependence receptor functionality of DCC may not be conserved in Drosophila , as the D1290 residue important for the apoptotic response [16] is not conserved in Fra and loss of fra in imaginal discs does not protect cells from apoptosis, but has the opposite effect [17] . To further characterize eversion defects, we imaged netA-IR pupae live using the His2Av-eGFP (enhanced green fluorescence protein) nuclear marker. Time-lapse sequences of netA-IR pupae showed a range of behaviours that corresponded to adult phenotypes with single ( n =2/12) and double ( n =4/12) eversion failure ( Fig. 1j,k ) and delayed or mismatched thoracic closure ( n =4; Fig. 1i ; Supplementary Movies 1–4 ). Before eversion, netA-IR wing discs appeared normal in position, size and morphology, and the behaviour of the polyploid epidermal cells throughout the eversion process was comparable to wild-type controls ( Fig. 1h ). Double-eversion failure was more commonly observed in pupae analysed by time-lapse microscopy than in adults examined for eversion defects, so this type of eversion failure appears to result in early pupal lethality. Mild adult phenotypes, such as thoracic clefts and missing/crumpled wings, are also likely to be due to a partial disruption of eversion, as similar phenotypes occur when the breakdown of the basement membrane is inhibited by expression of Tissue inhibitor of metalloproteases , which would disrupt the peripodial cells breaking through the overlying epidermis [8] . Pupae hemizygous for the classical double-mutant allele netAB Δ (ref. 18 ) were pupal lethal. However, when dissected at 4.5 h after puparium formation, a stage when eversion would normally have already taken place, netAB Δ pupae exhibited internalized wing discs in 35.3% ( n =17; Fig. 1f ) of progeny, similar to the defects seen in live netA-IR pupae. To determine whether eversion defects were simply due to a failure to activate the JNK pathway, we checked the expression of two JNK targets/reporters, puc-lacZ [19] and MMP1 (ref. 8 ), but both of these appeared normal ( Fig. 2a–f ). We also confirmed that NetA and Fra expression were not regulated by the JNK pathway, by checking expression of both proteins in discs hemizygous for hep R75 , a strong loss of function mutant for the JNK kinase hemipterous . Both appeared normal ( Fig. 2g–l and see below). These results identify the Netrins, particularly NetA, as new factors required for wing disc eversion. 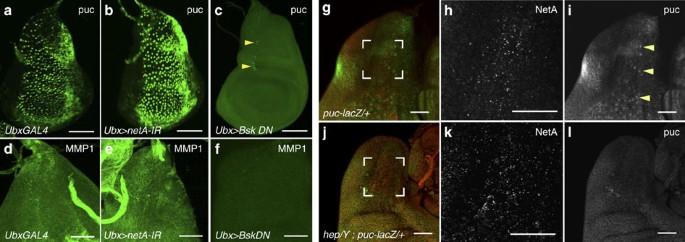Figure 2: The JNK pathway is activated innetA-IRdiscs and does not regulate NetA. (a–f) JNK pathway activity assessed by expression of two JNK targets,puc-lacZ(anti-β-gal,a–c) and anti-MMP1 (d–f). lacZ is expressed inUbx-GAL4, puc-lacZcontrol disc andUbx>netA-IR, puc-lacZdisc (b) but is lost inUbx>bskDN, puc-lacZdiscs (c) (although some lacZ expression persists outside theUbx-GAL4expression domain—arrowheads). Punctate anti-MMP1 staining was observed in the stalk region of controlUbx-GAL4/+(d), andUbx>netA-IR(e) third instar discs, but not inUbx>bskDNdiscs (f). (g–i) ControlUbx-GAL4, puc-lacZ/+ disc showing expression of NetA puncta (h) andpuc-lacZin peripodial cells (i, arrowheads). (j–l) InhepR75/Y;Ubx-GAL4,puc-lacZ/+ discs,puc-lacZexpression is lost (l), but NetA expression appears normal (k). Scale bars, 50 μm (a–c,g–l) and 10 μm (d–f). Figure 2: The JNK pathway is activated in netA-IR discs and does not regulate NetA. ( a – f ) JNK pathway activity assessed by expression of two JNK targets, puc-lacZ (anti-β-gal, a – c ) and anti-MMP1 ( d – f ). lacZ is expressed in Ubx-GAL4, puc-lacZ control disc and Ubx>netA-IR, puc-lacZ disc ( b ) but is lost in Ubx>bsk DN , puc-lacZ discs ( c ) (although some lacZ expression persists outside the Ubx-GAL4 expression domain—arrowheads). Punctate anti-MMP1 staining was observed in the stalk region of control Ubx-GAL4/+ ( d ), and Ubx>netA-IR ( e ) third instar discs, but not in Ubx>bsk DN discs ( f ). ( g – i ) Control Ubx-GAL4, puc-lacZ /+ disc showing expression of NetA puncta ( h ) and puc-lacZ in peripodial cells ( i , arrowheads). ( j – l ) In hep R75 /Y;Ubx-GAL4,puc-lacZ /+ discs, puc-lacZ expression is lost ( l ), but NetA expression appears normal ( k ). Scale bars, 50 μm ( a – c , g – l ) and 10 μm ( d – f ). Full size image netA regulates ZA breakdown in the peripodial epithelium Eversion defects could arise from a failure in the dissociation of the peripodial epithelium, a failure to breakdown the basement membrane and/or a failure to invade and migrate. To clarify which stage of eversion required netA and to more clearly image peripodial cells at the time of the epithelial dissociation, we isolated wing discs from third instar larvae and induced them to undergo eversion in culture medium using the moulting hormone ecdysone [10] , [20] . With this protocol, the peripodial epithelium breaks apart at around 7–8 h, and retracts back over the disc proper, eventually forming a clump of cells at the base of the exposed wing blade ( Fig. 3a,b ) [10] . When cultured for 24 h control Ubx>GFP , wing discs successfully everted in 81.25% ( n =96) of cases compared with only 60.75% ( n =107) for netA-IR discs ( Fig. 3c )—a significant reduction of 20.5% ( P =0.0019, Fisher’s exact test). Similarly, the netAB Δ /Y disc eversion rate (53.5%, n =71) was significantly lower than that of sibling control discs (that is, with one wild-type copy of the netrins; 78.38%, n =74; P =0.0026, Fisher’s exact test), and these values were not significantly different from netA-IR discs ( P =0.3562, Fisher’s exact test) and Ubx>GFP control discs ( P =0.7008, Fisher’s exact test) ( Fig. 3c ). 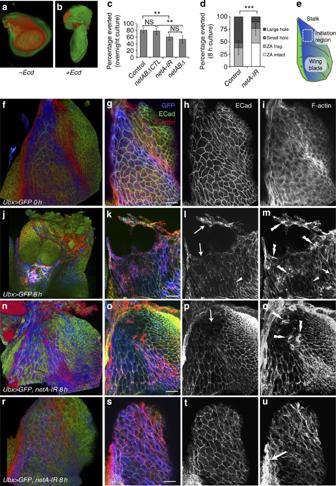Figure 3: NetA is required for eversion of the peripodial epithelium. (a,b) Third instar controlUbx>GFPdiscs cultured overnight without (a) or with ecdysone (b). Peripodial cells expressing GFP are shown in red. (c) Quantification of overnight eversion inUbx>GFP(control;n=96),netA-IR(n=107),netABΔ/Y(n=71) and netABΔsibling control discs (n=74) cultured in the presence of ecdysone (**=P<0.01; NS=P>0.05; Fisher’s exact test). (d) Quantification of eversion outcomes forUbx>GFP(control;n=40) andnetA-IR(n=47) discs after culturing for 8 h in ecdysone. Error bars are for the proportion with no holes (***=P<0.001; Fisher’s exact test). (e) Schematic representation of a third instar wing disc showing the Ubx expression domain (blue) and the ‘initiation region’. (f–u) Third instarUbx>GFP(control;f–m) andnetA-IR(n–u) wing discs cultured for 0 h (f–i) and 8 h (j–u), stained for F-actin (red inf,g,j,k,n,o,r,s) and E-Cad (green inf,g,j,k,n,o,r,s). Discs are shown as three-dimensional renderings (f,j,n,r) and maximum projections (g–i,k–m,o–q,s–u; see Methods andSupplementary Movie 5for image projection method). Scale bars, 20 μm (g,k,o,s). Error bars=95% confidence interval (Wilson score method). Figure 3: NetA is required for eversion of the peripodial epithelium. ( a , b ) Third instar control Ubx>GFP discs cultured overnight without ( a ) or with ecdysone ( b ). Peripodial cells expressing GFP are shown in red. ( c ) Quantification of overnight eversion in Ubx>GFP (control; n =96), netA-IR ( n =107), netAB Δ /Y ( n =71) and netAB Δ sibling control discs ( n =74) cultured in the presence of ecdysone (**= P <0.01; NS= P >0.05; Fisher’s exact test). ( d ) Quantification of eversion outcomes for Ubx>GFP (control; n =40) and netA-IR ( n =47) discs after culturing for 8 h in ecdysone. Error bars are for the proportion with no holes (***= P <0.001; Fisher’s exact test). ( e ) Schematic representation of a third instar wing disc showing the Ubx expression domain (blue) and the ‘initiation region’. ( f – u ) Third instar Ubx>GFP (control; f – m ) and netA-IR ( n – u ) wing discs cultured for 0 h ( f – i ) and 8 h ( j – u ), stained for F-actin (red in f , g , j , k , n , o , r , s ) and E-Cad (green in f , g , j , k , n , o , r , s ). Discs are shown as three-dimensional renderings ( f , j , n , r ) and maximum projections ( g – i , k – m , o – q , s – u ; see Methods and Supplementary Movie 5 for image projection method). Scale bars, 20 μm ( g , k , o , s ). Error bars=95% confidence interval (Wilson score method). Full size image To understand the cellular basis of eversion failure in netA-IR discs, we examined two key features of cells undergoing the EMT-like process at the onset of disc eversion, the breakdown of the ZA and rearrangements of the F-actin cytoskeleton [1] . In control discs at the start of the culturing period, E-Cad was localized to a thin, continuous, circumferential ZA ( Fig. 3f,g ). After 8 h culturing, in 52.5% of control discs ( n =40; Fig. 3d ) the peripodial epithelium had retracted leaving a large hole. In 10% of discs a smaller perforation had formed near the stalk ( Fig. 3d,j–m ). In these discs, both E-Cad and F-actin showed a graded distribution. In cells away from the perforation, E-Cad staining at the ZA remained intact ( Fig. 3l ; arrowhead). In these cells, F-actin appeared mostly coincident with E-Cad in the ZA ( Fig. 3m ; arrowhead) but also formed fibres within the cytoplasm ( Fig. 3m ; arrow). In cells closer to the hole, the ZA E-Cad became increasingly fragmented and delocalized ( Fig. 3l ; arrows) and cells showed strong aggregations of F-actin ( Fig. 3m ; double-arrowheads). In the remaining 37.5% of control discs, the epithelium was still intact but a similar fragmentation of E-Cad and enrichment of F-actin was seen in that region of the disc in which the holes usually formed. We will refer to this region, lying between the stalk and the first fold of the disc proper, and adjacent to the sharp border of Ubx expression as the ‘initiation region’ ( Fig. 3e ). In netA-IR discs cultured for 8 h, eversion was inhibited, with only 10.6% ( n =47) having large holes, 12.8% having small holes and 76.6% an intact peripodial epithelium, a significant difference from control discs ( P =0.004, Fisher’s exact test; Fig. 3d ). In 53.4% of discs (including all discs with holes), the delocalization of E-Cad ( Fig. 3p , arrow) and enrichment of F-actin ( Fig. 3q , double-arrowheads) appeared similar to control discs. In the remaining 46.8% of discs, however, the ZA E-Cad remained intact in the initiation region ( Fig. 3r–u ), a proportion similar to that of adult progeny with eversion defects. Interestingly, F-actin enrichment was still evident, particularly in that part of the initiation region closer to the sharp border of Ubx expression ( Fig. 3u ; arrow). Thus, F-actin enrichment is genetically separable from ZA fragmentation. As the JNK pathway is activated in netA-IR discs, this may be due to upregulation of targets such as the F-actin polymerization regulator chickadee (that is, Drosophila profilin) [21] . The results suggest that netA-IR eversion defects are due to a failure in the breakdown of the peripodial cell–cell junctions. Fra has an inhibitory role in eversion A key receptor of Drosophila Netrins is Fra. Fra is a well-known axon guidance receptor [22] but may also act as an epithelial maintenance factor. In eye-antennal discs, fra mutant clones, when rescued from death, display loss of epithelial polarity, increased pJNK and MMP1 expression, and increased invasiveness [17] . We speculated therefore that Fra might inhibit peripodial epithelial dissociation. Consistent with this, RNAi knockdown of fra , using four independent RNAi constructs, did not disrupt eversion ( Table 1 ), whereas Fra overexpression resulted in thoracic clefting and uneverted wings in 8.7% ( n =115) of progeny ( Fig. 4a,b ; Table 1 ). As for netA RNAi, these phenotypes were not affected by the co-expression of p35 ( Fig. 4k ). Although fra RNAi did not result in adult eversion phenotypes, we found that it was able to accelerate the epithelial dissociation of cultured wing discs. After 7 h of culturing, the proportion of discs in which ZA fragmentation had commenced was doubled from 33.3% ( n =18) in control discs to 65.2% ( n =23), and discs with holes increased from 5.5% to 13.0% ( Fig. 4l ). The lack of adult phenotypes associated with fra RNAi may be because early onset of eversion does not create defects that are apparent at adult stages. Alternatively, early onset of epithelial breakdown may not, on its own, lead to eversion in vivo , because other coordinated processes are required (for example, increases in MMPs), the timing of which is not altered by fra RNAi treatment. 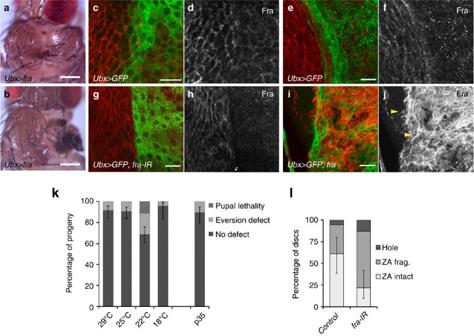Figure 4: Fra antagonizes disc eversion. (a,b)Ubx>fraadults displayed thoracic clefting (a) and eversion failures (b). (c–j) Anti-Fra immunostaining (red inc,e,g,i) of early (c–d) and late (e–j) third instar wing discs (see Methods for staging). Peripodial cells (marked withUbx>GFP—green) are to the right and disc proper cells to the left. (c–j) Fra expression inUbx>GFP(control),Ubx>GFP, fra-IR(g,h) andUbx>GFP, fra(i,j) third instar wing discs. (Note: exposure levels iniandjare reduced with respect to panelsc–h). (k) Penetrance of defects generated byfraoverexpression at various temperatures. For each genotype,n>40 progeny were scored (Table 1). (l) Quantification of eversion outcomes forUbx>GFP(control;n=18) andfra-IR(n=23) discs after culturing for 7 h in ecdysone. Scale bars, 200 μm (a,b) and 10 μm (c–i). Error bars=95% confidence interval (Wilson score method;k,l). Figure 4: Fra antagonizes disc eversion. ( a , b ) Ubx>fra adults displayed thoracic clefting ( a ) and eversion failures ( b ). ( c – j ) Anti-Fra immunostaining (red in c , e , g , i ) of early ( c – d ) and late ( e – j ) third instar wing discs (see Methods for staging). Peripodial cells (marked with Ubx>GFP —green) are to the right and disc proper cells to the left. ( c – j ) Fra expression in Ubx>GFP (control), Ubx>GFP, fra-IR ( g , h ) and Ubx>GFP, fra ( i , j ) third instar wing discs. (Note: exposure levels in i and j are reduced with respect to panels c – h ). ( k ) Penetrance of defects generated by fra overexpression at various temperatures. For each genotype, n >40 progeny were scored ( Table 1 ). ( l ) Quantification of eversion outcomes for Ubx>GFP (control; n =18) and fra-IR ( n =23) discs after culturing for 7 h in ecdysone. Scale bars, 200 μm ( a , b ) and 10 μm ( c – i ). Error bars=95% confidence interval (Wilson score method; k , l ). Full size image Next, Fra localization was assessed in peripodial cells before the epithelial dissociation. In late third instar discs, Fra localization differed between the peripodial and disc proper epithelia. In disc proper cells, Fra was enriched around the cell perimeter. This staining was not tightly localized to a thin cell–cell border but rather was somewhat diffuse, mottled and punctate ( Fig. 4e,f ). In peripodial cells, Fra did not outline cells but was instead localized to cytoplasmic puncta distributed evenly throughout the cell, and appeared reduced in levels ( Fig. 4f ). Fra expression was significantly diminished by RNAi, confirming the specificity of the staining ( Fig. 4g,h ). When Fra was overexpressed, cytoplasmic puncta were still present but Fra appeared more associated with the cell surface and cells exhibited extensive protrusions ( Fig. 4i,j , arrowheads), suggesting that the Fra signalling pathways that regulate cell motility become activated when Fra is expressed at high levels. We speculated therefore that more modest increases in Fra levels, such as those that occur in netA-IR discs (see below), might more effectively block eversion. To test this, we reduced expression levels by decreasing the temperature (the GAL4/UAS system being temperature dependent [23] ). At 22 °C, eversion defects were significantly increased to 20.1% ( n =159) and pupal lethality increased from 0 to 11.3% ( Fig. 4k , Table 1 ). At 18 °C, when GAL4 activity is low, eversion rates were reduced again. These results suggest that the response of peripodial cells is sensitive to Fra levels; at low levels epithelial dissociation occurs, at medium levels epithelial dissociation is inhibited and at higher levels cell motility is activated. Fra localization was also developmentally regulated. In early third instar discs, Fra localization was less punctate and more associated with the perimeter of peripodial cells, similar to disc proper cells ( Fig. 4c,d ). Thus, the loss of Fra from the cell perimeter correlates with the timing of the epithelial dissociation. Fra downregulation is NetrinA- and proteasome dependent NetA was also expressed in puncta in peripodial cells ( Fig. 5a–d ). In netA-IR discs, NetA puncta were significantly reduced in the peripodial cells ( Fig. 5e–h ) again confirming the specificity of the staining and showing that the NetA protein detected in peripodial cells is predominantly produced by the peripodial cells themselves. NetB was also expressed in a similar puncate pattern in peripodial cells ( Fig. 5i–l ). 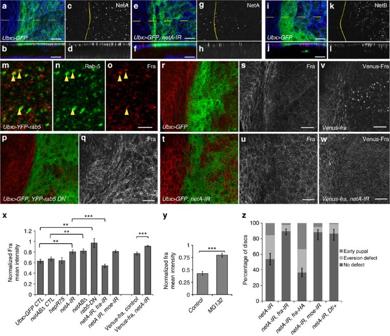Figure 5: Fra is endocytosed and degraded in a NetA-dependent manner to promote eversion. (a–u) ControlUbx>GFP(a–d,i–l,r,s),Ubx>netA-IR(e–h,t–u), Ubx>YFP-rab5(m–o) andUbx>YFP-rab5DNwing discs (p–q) stained for NetA (red,a,b,e,f), NetB (red,i,j), E-Cad (blue,a,b,e,f,i,j) and Fra (red,m–o,r,p,t).Ubx>CD8-GFP(green) marks peripodial cells. Yellow lines inc,gandkrepresent border of GFP expression. Dashed yellow lines ina,eandiindicate lines of cross-section depicted in panelsb,fandj, respectively. (v–w) Venus-Fra expression invenus-fra(v) andvenus-fra,netA-IR (w) discs (detected by anti-GFP immunostaining). (x) Mean intensity levels for Fra and Venus-Fra in peripodial cells relative to adjacent disc proper cells.N-values are Ubx>GFP (n=18),netABΔCTL(n=21),hepR75/Y(n=17),netA-IR(n=42),netABΔ/Y(n=37),Ubx>YFP-rab5DN(n=20),Ubx>netA-IR, fra-IR(n=15),Ubx>netA-IR, moe-IR(n=14), venus-fra(n=10), venus-fra; Ubx>netA-IR(n=9); (**P<0.01; ***P<0.001; Student’st-test). (y) Mean Fra intensity, relative to disc proper, in peripodial cells after 5 hin vitroculture at 25°C in the absence (n=11) or presence (n=13) 10 μM MG132 (***P<0.001; Student’st-test). (z) Quantification ofnetA-IRadult eversion defects when co-expressed withfra-IR,fra-HA,moe-IRand with heterozygosity forDf(2R)BSC880(which deletesfra). Scale bars, 10 μm (a–k,r–w) and 2.5 μm (m–o). Error bars=s.e.m. (x,y) and 95% confidence interval (Wilson score method;z). Figure 5: Fra is endocytosed and degraded in a NetA-dependent manner to promote eversion. ( a – u ) Control Ubx>GFP ( a – d , i – l, r , s ), Ubx>netA-IR ( e – h , t – u ), U bx>YFP-rab5 ( m – o ) and Ubx>YFP-rab5 DN wing discs ( p – q ) stained for NetA (red, a , b , e , f ), NetB (red, i , j ), E-Cad (blue, a , b , e , f , i , j ) and Fra (red, m – o , r , p , t ). Ubx>CD8-GFP (green) marks peripodial cells. Yellow lines in c , g and k represent border of GFP expression. Dashed yellow lines in a , e and i indicate lines of cross-section depicted in panels b , f and j , respectively. ( v – w ) Venus-Fra expression in venus-fra ( v ) and venus-fra ,netA-IR ( w ) discs (detected by anti-GFP immunostaining). ( x ) Mean intensity levels for Fra and Venus-Fra in peripodial cells relative to adjacent disc proper cells. N -values are Ubx>GFP ( n =18), netAB Δ CTL ( n =21), hep R75 /Y ( n =17), netA-IR ( n =42), netAB Δ /Y ( n =37), Ubx>YFP-rab5 DN ( n =20), Ubx>netA-IR, fra-IR ( n =15), Ubx>netA-IR, moe-IR ( n =14) , venus-fra ( n =10) , venus-fra; Ubx>netA-IR ( n =9); (** P <0.01; *** P <0.001; Student’s t -test). ( y ) Mean Fra intensity, relative to disc proper, in peripodial cells after 5 h in vitro culture at 25°C in the absence ( n =11) or presence ( n =13) 10 μM MG132 (*** P <0.001; Student’s t -test). ( z ) Quantification of netA-IR adult eversion defects when co-expressed with fra-IR , fra-HA , moe-IR and with heterozygosity for Df(2R)BSC880 (which deletes fra ). Scale bars, 10 μm ( a – k , r – w ) and 2.5 μm ( m – o ). Error bars=s.e.m. ( x , y ) and 95% confidence interval (Wilson score method; z ). Full size image A proportion of the Fra puncta in late third instar discs co-localized with the early endosome marker YFP-Rab5 ( Fig. 5m–o ) suggesting that Fra-positive puncta were associated with endocytic vesicles. Further, expression of a dominant-negative YFP-Rab5 S43N transgene [24] increased the levels of cytoplasmic Fra staining, such that the darker nuclear region was more apparent ( Fig. 5p,q ) than in control discs ( Fig. 5r,s ). As Rab5 is required for early endosome formation [25] , [26] this suggests that the reduction in Fra levels involves an endocytic pathway. We quantified the increase in Fra by normalizing mean intensity in peripodial cells to mean intensity in an adjacent region of disc proper cells (see Methods). Fra levels were significantly increased from 0.628 ( n =18) in control discs to 0.968 ( n =20) in Ubx>YFP-Rab5 S43N discs ( P =0.0041, Student’s t -test; Fig. 5x ). These pupae died early in pupal development, and on dissection all progeny displayed eversion defects. We also checked Fra levels in hep R75 /Y discs and found the results were non-significantly different from Ubx>GFP control discs (0.639, n =17, P =0.852, Student’s t -test, Fig. 5x ). Downregulation of receptors via ligand-mediated receptor endocytosis and lysosomal degradation is a common cellular mechanism [27] , [28] . In vertebrates, the DCC receptor is endocytosed and degraded via a ubiquitin–proteasome pathway on binding Netrin-1 (refs 29 , 30 ), a mechanism thought to regulate growth cone responses to Netrin-1 (refs 31 , 32 ). We therefore tested whether Fra levels were regulated by NetA and by the proteasome. As expected, Fra levels were significantly increased in netA-IR discs ( Fig. 5t,u ) to 0.802 ( n =42; P <0.001, Student’s t -test; Fig. 5x ). Similarly, Fra levels in netAB Δ /Y discs were (0.818, n =37), which were significantly higher than sibling control discs (0.672, n =21; P =0.012, Student’s t -test), and these values were not significantly different from netA-IR discs ( P =0.716, Student’s t -test) and Ubx>GFP control discs ( P =0.396, Student’s t -test) ( Fig. 5x ). As an independent way of assessing the effect of netA RNAi on Fra levels, we utilized an exon trap line in which the coding sequence of the venus gene is spliced into the frazzled gene, between the amino-terminal signal sequence and the first extracellular IgG domain. In venus-fra/+ control discs, Venus-Fra was expressed in a similar punctate pattern to endogenous Fra and, similar to endogenous Fra, was reduced in peripodial cells relative to the disc proper cells ( Fig. 5v,x ), and levels were increased when netA-IR was expressed ( Fig. 5w,x ). Next, we cultured discs for 5 h in the presence of the proteosome inhibitor MG132. Fra levels were significantly elevated with respect to control discs, from 0.427 ( n =11) to 0.799 ( n =13; Fig. 5y ; P <0.0001, Student’s t -test). Thus, as in vertebrates, Netrin promotes the downregulation of the Fra receptor, and this probably depends on the proteasome. Interestingly, the endocytosis of Fra seemed to be independent of NetA, as Fra puncta were present in both disc proper cells, where NetA levels are low, and in peripodial cells of netA-IR discs. We next tested whether the increase in Fra levels in net-IR discs could account for the eversion defects. Importantly, fra RNAi in netA-IR discs substantially rescued the eversion phenotypes, with the proportion of unaffected progeny increasing from 53.9 to 89.4% ( n =292, Fig. 5z ), and restored peripodial Fra levels to a value similar to control discs of 0.540 ( n =15, P <0.001, Student’s t -test; Fig. 5x ). Eversion defects could also be suppressed by heterozygosity for the deficiency Df(2R)BSC880, which removes fra (86.5% normal progeny, n =89; Fig. 5z ). Thus, netA-IR eversion defects are largely due to excess Fra. Moe acts downstream of Fra in opposing eversion Finally, we sought to determine the downstream pathway by which Fra might inhibit epithelial dissociation. One factor known to maintain epithelial integrity in flies is the ERM-family protein, Moe. Loss of moe in wing disc epithelia results in the loss of polarity and adhesion, and acquisition of motile and invasive behaviours [33] . Further, in vertebrates DCC binds to the ERM-family protein Ezrin and can regulate its phosphorylation [34] . We therefore tested levels of Moe activation (using an antibody that recognizes phosphorylated Moe) to see whether they correlated with Fra expression. p-Moe staining showed similar expression patterns to Fra, in that it was punctate and reduced in wild-type peripodial cells with respect to the disc proper ( n =15; Fig. 6a,b ) and was significantly increased by RNAi knockdown of netA ( n =17, P =0.0011, Student’s t -test; Fig. 6c,d,g ). This increase was specific to the phosphorylated form of Moe, as an antibody that detects total Moe showed no significant difference in levels between peripodial cells and disc proper cells, in either control or netA-IR discs ( Fig. 6h ). Overexpression of Fra also increased p-Moe levels ( n =23, P =0.025, Student’s t -test; Fig. 6e–g ), although levels were comparable to those in Ubx>netA-IR discs suggesting a rate-limiting component in the pathway by which Fra activates Moe. Most importantly, netA-IR eversion defects were almost completely suppressed by moe RNAi ( n =153; Fig. 5z and Table 1 ), although Fra levels remained high (no significant difference compared with netA-IR; Fig. 5x ) suggesting that it is the activation of Moe that blocks epithelial dissociation, rather than the increase in Fra. Finally, p-Moe staining was significantly decreased in Ubx>netA-IR,fra-IR discs ( n =14, P =0.0018, Student’s t -test; Fig. 6g ) compared with netA-IR discs showing that Fra is required for Moe activation. Expression of moe , moe T559D or moe T559A transgenes did not cause eversion defects, however, suggesting that Moe is necessary but not sufficient for the inhibition of epithelial dissociation. Alternatively, the phosphorylated form of Moe seen in netA-IR discs may have post-translational modifications, in addition to the phosphorylation at T559, that are important in blocking the epithelial dissociation. On the basis of these results, we propose a model in which Fra-dependent activation of Moe promotes an epithelial state, and NetA promotes epithelial dissociation by downregulating Fra. 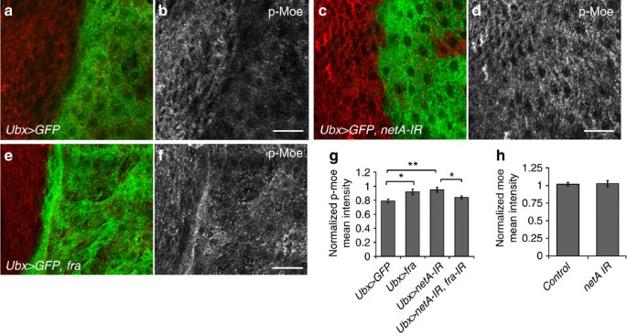Figure 6: Fra promotes Moe phosphorylation. (a–f) Anti-phospho-Moe staining (red,a,c,e) inUbx>GFP(control;a,b),netA-IR(c,d)and Ubx>fra(e,f) discs. (g) Quantification of mean intensity levels for p-Moe in peripodial cells relative to adjacent disc proper cells.N-values areUbx>GFP/+(n=15),Ubx>fra(n=23),Ubx>netA-IR(n=17),Ubx>netA-IR, fra-IR(n=14); (*P<0.05; **P<0.01; Student’st-test). (h) Mean intensity levels for Moe in peripodial cells were comparable to adjacent disc proper cells in control (n=8) andnetA-IR(n=6) discs. Scale bars, 10 μm (a–f). Error bars=s.e.m. (g) and 95% confidence interval (Wilson score method;h). Figure 6: Fra promotes Moe phosphorylation. ( a – f ) Anti-phospho-Moe staining (red, a , c , e ) in Ubx>GFP (control; a , b ), netA-IR ( c , d ) and Ubx>fra ( e , f ) discs. ( g ) Quantification of mean intensity levels for p-Moe in peripodial cells relative to adjacent disc proper cells. N -values are Ubx>GFP/+ ( n =15), Ubx>fra ( n =23), Ubx>netA-IR ( n =17), Ubx>netA-IR, fra-IR ( n =14); (* P <0.05; ** P <0.01; Student’s t -test). ( h ) Mean intensity levels for Moe in peripodial cells were comparable to adjacent disc proper cells in control ( n =8) and netA-IR ( n =6) discs. Scale bars, 10 μm ( a – f ). Error bars=s.e.m. ( g ) and 95% confidence interval (Wilson score method; h ). Full size image Our results delineate a novel regulatory mechanism controlling wing disc eversion in which a Fra–Moe pathway required for maintenance of epithelial adhesion junctions is inhibited by Netrin-dependent degradation of the receptor. The Netrin/Fra pathway appears to act in parallel to the JNK pathway, as loss of netA did not prevent JNK activation and loss of JNK activation did not affect Fra or NetA levels. Given the intermediate penetrance of netA-IR phenotypes, the reduction of Fra must be only one of several redundant mechanisms required for eversion. The idea that Fra may act as an epithelial maintenance factor is supported by recent findings from our own laboratory in which loss of netrins or fra causes defects in the formation of the embryonic midgut epithelium (Pert et al. , unpublished observations). In vertebrates, DCC expression in epithelia has been reported for a variety of tissues such as the skin, gut, lung and bladder [35] , and DCC has been shown to increase cell–cell adhesion in both HT-29 cells [36] and fibroblasts [35] . Given the punctate distribution of Fra in netA-IR discs, its ability to stabilize the ZA is presumably not through some structural or adhesive role at the ZA but rather via signalling from endosomes. Elucidating the molecular pathway linking Fra, Moe and ZA maintenance, and understanding how that pathway interacts with molecular processes acting downstream of JNK activation (such as MMP breakdown of the basement membrane) are important future goals. The opposing roles for NetA and Fra demonstrated here correlate with previous descriptions of Netrin-1 as an oncogene [37] and DCC as a tumour suppressor [16] . Netrin-1 levels are elevated in metastatic breast cancers [37] and strongly overexpressed in human pancreatic cancer [38] . Further, overexpression of Netrin-1 is associated with tumour formation and progression in mice [12] , whereas in mammary metastatic tumour cell lines, metastatic progression was blocked when Netrin-1 expression was decreased [37] . Although current research focuses largely on the role of DCC as a dependence receptor (reviewed in ref. 39 ) the effects of increased Netrin-1 or decreased DCC expression on cells at early stages of metastasis are unclear. The findings from this study raise the possibility that Netrins may not only promote cell migration and the subsequent survival of metastasized cells but also influence the initial loss of the epithelial state. Drosophila stocks The following fly stocks were used in this study: Ubx-GAL4 (ref. 40 ), netABΔ (ref. 18 ), UAS-netA and UAS-netB [15] . The following strains were obtained from the Bloomington Drosophila Stock Center at Indiana University: UAS-fra, UAS-YFP-rab5 DN , UAS-YFP-rab5, puc E69 , UAS-Bsk DN , UAS-p35, His2Av-eGFP, UAS-mCD8-GFP and hep R75 . venus-Fra [ CPTI-001309 ] ( http://www.flybase.org/reports/FBal0262139.html ) was obtained from the Drosophila Genetics Resource Centre. All UAS-RNAi stocks were obtained either from the Vienna Drosophila RNAi Centre or the Bloomington Stock Centre. The following stocks were made in this study: Ubx-GAL4,UAS-mCD8-GFP, Ubx-GAL4,puc-lacZ, His2AvGFP;Ubx-GAL4, UAS-p35;Ubx-GAL4, UAS-fra;Ubx-GAL4 and venus-Fra;Ubx-GAL4 . netAB Δ control larvae were those with one copy of the FM7 kr>GFP balancer (that is, the viable genotype), which were readily distinguished from the FM7 kr>GFP / FM7 kr>GFP females by the brightness of the GFP signal. Pupal live imaging Laser confocal microscopy was used to capture live images of His2AvGFP pupae through the pupal case. Pupae were mounted by adhering the operculum to a cover glass with a drop of liquid paraffin. An inverted SP5 Leica confocal microscope was used in a room that was maintained at ~25 °C. Exact settings varied with experiment but were chosen to balance the need for a clear image with minimizing laser exposure to avoid tissue damage. Typically, 7–15 z -sections with a 3-μm step size were captured every 60–90 s with a × 20 lens. In vitro disc culture In vitro disc culture was essentially as described [10] . Third instar wandering larvae were rinsed in PBS buffer and then dissected in culture medium (Shields and Shang M3 medium, Sigma (S3652) supplemented with 2% FCS, 0.5% penicillin–streptomycin (15140–122; Invitrogen) and 20-hydroxyecdysone (Sigma, H5142) at a final concentration of 0.2 μg ml −1 ). Fat body and gut were removed. Culturing was performed in glass cavity blocks kept at 25 °C in a humidified chamber. Discs were dissected out of multiple larvae over a period of ~20–30 min such that timed-culturing periods are accurate to within ±15 min. Subsequent fixation and staining was performed using standard methods. For analysis of discs in which the protesasome was inhibited, discs were cultured for 5 h at 25 °C before fixation and staining. For treatment with MG132 (Sigma, C2211), discs were cultured in medium containing 40 μM MG132 (experimental discs) or an equivalent volume of dimethyl sulfoxide (control discs). Immunohistochemistry Two stages of third instar larvae were used in this study. Late third instar larvae correspond to wandering third instar larvae that had emerged from the food. Early third instar larvae were pulled from the food and their discs were on average ~25% smaller than late third instar larvae. Unless otherwise stated, all wing discs are from late third instar larvae. Wing imaginal discs were dissected out of third instar larvae and fixed in 4% formaldehyde in 1 × PBS for 20 min and washed in PBS, 0.1% Triton X-100. The following primary antibodies were used: rat anti-DE-Cadherin (DCAD2, Developmental Studies Hybridoma Bank (DSHB), 1:100), mouse anti-β-gal (40-1a-c DSHB, 1:100), mouse anti-MMP1 (3B8D12-c, 14A3D2-c, 5H7B11-c DSHB; antibodies were used in combination each at 1:100), mouse anti-GFP (GFP-G1 DSHB; 1:100), rabbit-anti-Phospho-Ezrin(Thr567)/Radixin (Thr564)/Moesin (Thr558; Cell Signalling, 1;100), rabbit-anti-Fra [22] (a gift from Florence Maschat, 1:250), rabbit anti-moesin (a gift from Dan Kiehart, 1:200) [41] and rabbit-anti-NetB [42] (a gift from B. Altenhein). NetA immunostains utilized a peptide antibody raised against residues 633–642 (unpublished; a gift from Ben Altenhein, 1:100). Secondary antibodies used were highly cross-absorbed varieties. Fluorescent Alexa-488, Alexa-568 (Invitrogen) or Dy649 (Jackson ImmunoResearch) were used at 1:200. For nuclear staining of pupal tissue, Hoechst 33258 (Sigma) was used at 20 μg ml −1 . To stain filamentous actin, tissues were incubated in 80 μm rhodamine phalloidin (Invitrogen) in PBS, 0.1% Triton X-100 for 2 h at room temperature or overnight at 4 °C. Image capture and analysis Light microscopy was performed on a Leica M165 FC stereomicroscope and images were collected digitally with a Leica IC80HD camera. Fluorescence microscopy was performed on a confocal microscope using either Leica SP2 system or the Olympus FV1000. All images were acquired taken at 1,024 × 1,024 pixels and ImageJ was used for all image preparation. To quantify Fra levels, we calculated the ratio of mean intensity (arbitrary units) between a region ~ 20 cells in size in the peripodial epithelium adjacent to the disc proper and an adjacent region of disc proper tissue. In peripodial cells, intensity measurements were made on an average projection of four slices of a z-stack (corresponding to a 1-μm-thick section) whose apical-most slice was coincident with the position of the E-Cad-positive ZA. To enable visualization of the thin peripodial epithelium without interference from the underlying disc proper epithelium, image processing was performed. For each slice in which there was a clear gap between the disc proper cells and the peripodial cells, a polygonal region was digitized between them and this region was subtracted from the original image. Supplementary Movie 5 shows the regions subtracted for each z-slice of the maximum intensity projection control image shown in Fig. 3k . Statistics Fisher’s exact test was used for comparison of proportions of categories in disc culture and adult eversion tests. Comparison of Fra and Moe mean intensity ratios used a two tailed, Student’s t -test. All 95% confidence intervals were calculated using the Wilson score method with no continuity correction. Statistical significance markers are as follows: * P <0.05, ** P <0.01, *** P <0.001. How to cite this article: Manhire-Heath, R. et al. Netrin-dependent downregulation of Frazzled/DCC is required for the dissociation of the peripodial epithelium in Drosophila . Nat. Commun. 4:2790 doi: 10.1038/ncomms3790 (2013).